A meta-analysis of Hodgkin lymphoma reveals 19p13.3TCF3as a novel susceptibility locus Recent genome-wide association studies (GWAS) of Hodgkin lymphoma (HL) have identified associations with genetic variation at both HLA and non-HLA loci; however, much of heritable HL susceptibility remains unexplained. Here we perform a meta-analysis of three HL GWAS totaling 1,816 cases and 7,877 controls followed by replication in an independent set of 1,281 cases and 3,218 controls to find novel risk loci. We identify a novel variant at 19p13.3 associated with HL (rs1860661; odds ratio (OR)=0.81, 95% confidence interval (95% CI)=0.76–0.86, P combined =3.5 × 10 −10 ), located in intron 2 of TCF3 (also known as E2A ), a regulator of B- and T-cell lineage commitment known to be involved in HL pathogenesis. This meta-analysis also notes associations between previously published loci at 2p16, 5q31, 6p31, 8q24 and 10p14 and HL subtypes. We conclude that our data suggest a link between the 19p13.3 locus, including TCF3 , and HL risk. Hodgkin lymphoma (HL) is an aetiologically and histologically heterogeneous disease characterized by the presence of rare malignant Hodgkin Reed–Sternberg (HRS) cells [1] . It is one of the most common cancers among young adults in Western countries [2] , [3] . Classical HL (cHL) makes up the vast majority of HL and itself comprises several subtypes. Nodular sclerosis HL (NSHL) is the most common subtype among adolescents and young adults and is typically Epstein–Barr virus (EBV) negative [4] , [5] , [6] . Mixed cellularity HL (MCHL) is more common among young children and older individuals and its tumour cells typically contain EBV (EBV-positive HL) [4] , [5] , [6] . HL has a strong genetic component, with a highly increased risk in monozygotic compared with dizygotic co-twins [7] and other siblings [8] of a case, whose risk in turn is several times higher than the risk to an average person. It has been demonstrated that HLA is strongly associated with the risk of HL and that associated loci vary by EBV tumour status, with EBV-positive cHL associated with HLA-A *01 and HLA-A *02 class I alleles, and EBV-negative cHL associated with markers in or near the HLA class II region [6] , [9] , [10] . Three independent HL genome-wide association studies (GWAS) in persons of European origin have recently been published; two included all patients with cHL [11] , [12] and one was limited to adolescent/young adult patients with NSHL [13] . The most significantly associated SNPs in all three GWAS were located at the 6p21.32 region, which contains the HLA genes. Multiple independent variants within this region were associated with HL, with heterogeneity based on EBV tumour status and histological subtype [11] , [12] , [13] . Non-HLA risk loci were also identified, including REL , GATA3 and IL13 , some of which showed heterogeneity by histological subtype or EBV subgroup [11] , [12] . These studies collectively do not explain all genetic susceptibility for HL. Here we perform a meta-analysis to identify additional variants associated with HL and to investigate shared and unique susceptibility loci for different HL histological subtypes and EBV status-stratified subgroups. This study is the largest to date for this disease, with 3,097 cases and 11,095 controls included in the combined discovery and replication sets. We note HL subtype-specific associations with previously reported SNPs and identify a new HL susceptibility locus at 19p13.3. The discovery set included 1,816 cases and 7,877 controls from three GWAS conducted at the following centres: University of Southern California (USC) [13] ; International Agency for Research on Cancer (IARC) [12] ; and University of Chicago (UC) [14] ( Fig. 1 , Supplementary Fig. 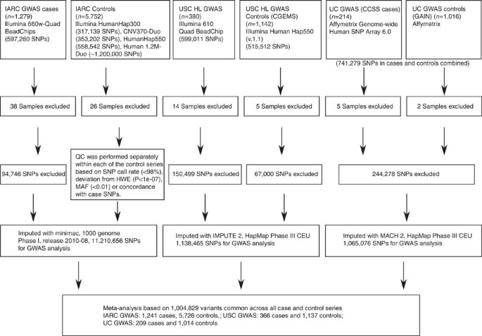Figure 1: Quality control for subjects and SNPs in the GWAS discovery meta-analysis. Details for each GWAS have been previously published12,13,14. 1 , Supplementary Table 1 ). Of the 1,816 cases, 58% were diagnosed between the ages of 15 and 35, 49% were female and 68% had HL tumours classified as NSHL. EBV tumour status was available for 1,063 cases; of these 27% were EBV positive. Fifty percent of the EBV-positive cases were MCHL. Conversely, 57% and 20% of MCHL and NSHL, respectively, were EBV positive, roughly similar to the distribution observed in a California population. [5] Adolescents and young adults aged 15–35 diagnosed with NSHL had the lowest proportion of EBV-positive tumours (17%), as expected. Figure 1: Quality control for subjects and SNPs in the GWAS discovery meta-analysis. Details for each GWAS have been previously published [12] , [13] , [14] . Full size image For the meta-analysis, we first applied quality control methods and imputation, which resulted in a total of 1,004,829 SNPs that were in common between the three studies ( Fig. 1 , Supplementary Fig. 2 (ref. 15 )). When considering the global GWAS results, there was some evidence of a general inflation of the test statistic ( λ =1.10, and excluding the MHC region, λ =1.09). However, after normalizing for sample size [16] , the degree of inflation was modest ( λ 1000 =1.03). The discovery meta-analyses of HL and subtypes were based on the 1,816 overall HL, 1,694 classical, 1,233 NSHL, 792 NSHL diagnosed between 15–35 years old, and 320 MCHL cases, each compared with the same 7,877 controls. Analyses stratified on EBV tumour status were based on 287 EBV-positive HL and 776 EBV-negative HL compared with 6,863 controls from the subset of studies with EBV testing ( Supplementary Table 1 ). The individual study results were combined using an inverse variance-weighted meta-analysis under the fixed effects model used to generate all P -values reported below for GWAS associations. 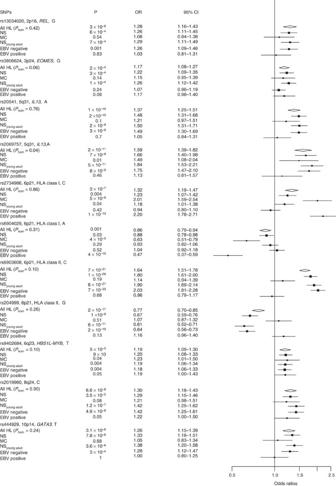Figure 2: Effect of genetic risk variants on the risk of Hodgkin lymphoma. Combined ORs and 95% CIs were derived from combining the three individual GWAS-specific estimates in a meta-analysis using a fixed-effect model. Individual GWAS estimates (OR and 95% CIs) were derived from the unconditional logistic regression adjusted for sex, study center (for European Collaborative GWAS only) and significant principal components, assuming additive model of inheritance.P-values for homogeneity between different subgroups were calculated using Cochran’sQ-statistic. Squares represent summary estimates; the size of the square represents inverse of the variance of the log ORs; horizontal lines represent 95% CIs; diamonds represent results for the total HL; solid vertical lines represent OR=1. Note that rs9402684 is substituted for rs7745098 (r2=0.90), which was not available in all three contributing GWAS. All HL, all subtypes of Hodgkin lymphoma combined (1,816 cases, 7,877 controls), NS, nodular sclerosis (1,233 cases, 7,877 controls), MC, mixed cellularity (320 cases, 7,877 controls), NSyoung, nodular sclerosis diagnosed in young adults 15–35 years old (792 cases, 7,877 controls), EBV negative (776 cases, 6,863 controls), EBV positive (287 cases, 6,863 controls). The meta-analysis revealed HL subtype-specific associations with genotypic variants at 2p16 ( REL ), 5q31 ( IL13 ), 6p21 (HLA), 8q24 and 10p14 ( GATA3 ) and the two recently described loci at 3p24 ( EOMES ) and 6q23 ( HBS1L-MYB ), consistent with previous reports [11] , [12] , [13] , [17] ( Figs 2 , 3 , Supplementary Table 2 (ref. 15 ), Supplementary Fig. 3 ). As expected, the SNPs near genes coding HLA class I alleles were strongly associated with EBV-positive HL and MCHL, but not EBV-negative HL or NSHL, while associations with SNPs near or in genes coding HLA class II alleles showed the opposite pattern ( Fig. 2 ). We identified two SNPs within the regions of 2p16 ( REL ) and 10p14 ( GATA3 ), rs13034020 ( P =3.2 × 10 −6 ) and rs444929 ( P =3.1 × 10 −6 ), in our analysis that were more significantly associated with HL than the previously reported SNPs rs1432295 and rs485411 (ref. 11 ) in these respective regions ( Supplementary Fig. 3 ). 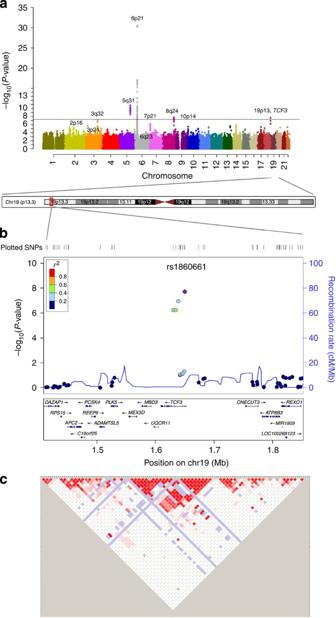Figure 3: Results of a meta-analysis of three GWAS of Hodgkin lymphoma. (a) Manhattan plot of genome-wide results of a case–control comparison of 1,816 Hodgkin lymphoma patients and 7,877 controls of European origin.P-values were determined for each SNP based on the overall meta-analysis using a fixed-effects model. Five loci surpassed the genome-wide significance level ofP=5 × 10−8, including four previously reported SNPs at 6p21 (HLA class II) and 5q31 (IL13) and one novel SNP (rs1860661 at 19p13.3) located inTCF3. Noteworthy loci from previous reports replicated here atP=≤0.05 are also shown, including those at 2p16 (REL), 3p24 (EOMES), 6q23 (HBS1L-MYB), 8q24 and 10p14 (GATA3), in addition to two novel loci at 3q32 (CLSTN2) and 7p21 (ARLA4-ETV1) from this meta-analysis that did not replicate. Note that data for rs7745098 at 6q23 were not available in all three contributing GWAS, thus data for rs9402684 atr2=0.90 was substituted. Variants withI2values⩾75% indicative of significant heterogeneity were excluded. (b) Regional plot of the 19p13.3 locus. Results (−log10P) are shown for SNPs genotyped and imputed within the region. The diamond represents the most significant SNP in the locus and ther2values for the other SNPs are indicated by different colours depending on the LD level in the CEU population. The genes within the region are annotated and shown as arrows. (c) Linkage disequilibrium map of the 19p13.3 locus (red representsr2>0.9). When conditioned on the previously reported SNPs, the association between HL and rs13034020 ( P =1.2 × 10 −3 ) and rs444929 ( P =1.8 × 10 −3 ) remained significant ( Supplementary Table 3 ). These SNPs, in addition to rs20541 in the IL13 gene region, were more strongly associated with EBV-negative HL and NSHL compared with EBV-positive and MCHL ( Fig. 2 , Supplementary Table 2 ). There was little difference in association by subtype/subgroup for the loci in the 3p24 and 6q23 regions ( Fig. 2 ). Figure 2: Effect of genetic risk variants on the risk of Hodgkin lymphoma. Combined ORs and 95% CIs were derived from combining the three individual GWAS-specific estimates in a meta-analysis using a fixed-effect model. Individual GWAS estimates (OR and 95% CIs) were derived from the unconditional logistic regression adjusted for sex, study center (for European Collaborative GWAS only) and significant principal components, assuming additive model of inheritance. P -values for homogeneity between different subgroups were calculated using Cochran’s Q -statistic. Squares represent summary estimates; the size of the square represents inverse of the variance of the log ORs; horizontal lines represent 95% CIs; diamonds represent results for the total HL; solid vertical lines represent OR=1. Note that rs9402684 is substituted for rs7745098 ( r 2 =0.90), which was not available in all three contributing GWAS. All HL, all subtypes of Hodgkin lymphoma combined (1,816 cases, 7,877 controls), NS, nodular sclerosis (1,233 cases, 7,877 controls), MC, mixed cellularity (320 cases, 7,877 controls), NSyoung, nodular sclerosis diagnosed in young adults 15–35 years old (792 cases, 7,877 controls), EBV negative (776 cases, 6,863 controls), EBV positive (287 cases, 6,863 controls). Full size image Figure 3: Results of a meta-analysis of three GWAS of Hodgkin lymphoma. ( a ) Manhattan plot of genome-wide results of a case–control comparison of 1,816 Hodgkin lymphoma patients and 7,877 controls of European origin. P -values were determined for each SNP based on the overall meta-analysis using a fixed-effects model. Five loci surpassed the genome-wide significance level of P =5 × 10 −8 , including four previously reported SNPs at 6p21 (HLA class II) and 5q31 ( IL13 ) and one novel SNP (rs1860661 at 19p13.3) located in TCF3 . Noteworthy loci from previous reports replicated here at P =≤0.05 are also shown, including those at 2p16 ( REL ), 3p24 ( EOMES ), 6q23 ( HBS1L-MYB ), 8q24 and 10p14 ( GATA3 ), in addition to two novel loci at 3q32 ( CLSTN2 ) and 7p21 ( ARLA4-ETV1 ) from this meta-analysis that did not replicate. Note that data for rs7745098 at 6q23 were not available in all three contributing GWAS, thus data for rs9402684 at r 2 =0.90 was substituted. Variants with I 2 values ⩾ 75% indicative of significant heterogeneity were excluded. ( b ) Regional plot of the 19p13.3 locus. Results (−log 10 P) are shown for SNPs genotyped and imputed within the region. The diamond represents the most significant SNP in the locus and the r 2 values for the other SNPs are indicated by different colours depending on the LD level in the CEU population. The genes within the region are annotated and shown as arrows. ( c ) Linkage disequilibrium map of the 19p13.3 locus (red represents r 2 >0.9). Full size image We found a novel susceptibility variant (rs1860661) surpassing the threshold for genome-wide significance located at chromosome 19p13.3 within intron 2 of the TCF3 gene (OR=0.78, P =2.0 × 10 −8 , I 2 =0%) ( Fig. 3 , Table 1 ). This variant was also significantly associated with all HL (OR=0.85, P =0.0024) in the replication series of 1,163 all HL cases and 2,580 controls of European descent ( Table 1 , Fig. 4 ). In the combined analysis, rs1860661 was strongly associated with all HL (OR=0.81, P =3.5 × 10 −10 ), with no evidence of statistically significant heterogeneity between contributing studies ( P hom=0.41, I 2 =0%). Inconsistent associations by histologic subtype (MCHL) and EBV status (EBV-positive HL) between the discovery and replication sets were likely to be chance findings due to small numbers ( Table 1 ). Table 1 The association of the G allele of SNP rs1860661* with risk of Hodgkin lymphoma by EBV subgroup and histological subset. 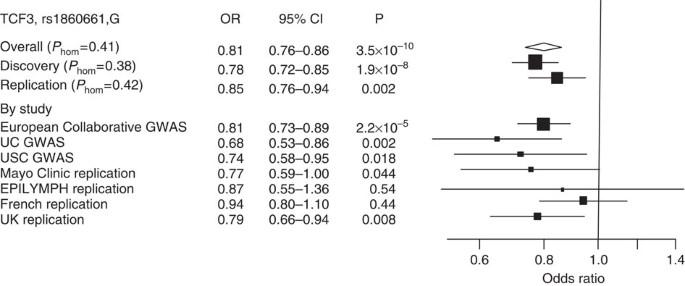Figure 4: Forest plot of discovery and replication ORs and 95% CIs for the association between 19p13.3TCF3rs1860661 and Hodgkin lymphoma by study. ORs and 95% CIs were derived from the unconditional logistic regression adjusted for sex and significant principal components (for individual GWAS analysis only), assuming additive model of inheritance. Squares represent ORs; the size of the square represents inverse of the variance of the log ORs; horizontal lines represent 95% CIs; diamonds represent summary estimate combining the study-specific estimates with a fixed-effects model; solid vertical lines represent OR=1; the dashed vertical line represents the overall OR.P-values for homogeneity between different subgroups were calculated using Cochran’sQ-statistic. Samples sizes are as follows: combined discovery and replication (3,097 cases and 11,095 controls); overall discovery (1,816 cases and 7,877 controls) consisted of European Collaborative GWAS (1,241 cases and 5,726 controls); USC GWAS (366 cases and 1,137 controls); UC GWAS (209 cases and 1,014 controls); overall replication (1,163 cases and 2,580 controls) consisted of Mayo Clinic (234 cases and 223 controls); EPILYMPH (64 cases and 141 controls); French Replication Series (LYSA/CNG Evry France) (366 cases and 1,696 controls); UK Replication Series (ELCCS (York)/Scotland and Newcastle Epidemiological Study of Hodgkin Disease (499 cases and 520 controls). The Scandinavian SCALE study is not included as rs1860661 could not be genotyped in controls using Sequenom. Full size table Figure 4: Forest plot of discovery and replication ORs and 95% CIs for the association between 19p13.3 TCF3 rs1860661 and Hodgkin lymphoma by study. ORs and 95% CIs were derived from the unconditional logistic regression adjusted for sex and significant principal components (for individual GWAS analysis only), assuming additive model of inheritance. Squares represent ORs; the size of the square represents inverse of the variance of the log ORs; horizontal lines represent 95% CIs; diamonds represent summary estimate combining the study-specific estimates with a fixed-effects model; solid vertical lines represent OR=1; the dashed vertical line represents the overall OR. P -values for homogeneity between different subgroups were calculated using Cochran’s Q -statistic. Samples sizes are as follows: combined discovery and replication (3,097 cases and 11,095 controls); overall discovery (1,816 cases and 7,877 controls) consisted of European Collaborative GWAS (1,241 cases and 5,726 controls); USC GWAS (366 cases and 1,137 controls); UC GWAS (209 cases and 1,014 controls); overall replication (1,163 cases and 2,580 controls) consisted of Mayo Clinic (234 cases and 223 controls); EPILYMPH (64 cases and 141 controls); French Replication Series (LYSA/CNG Evry France) (366 cases and 1,696 controls); UK Replication Series (ELCCS (York)/Scotland and Newcastle Epidemiological Study of Hodgkin Disease (499 cases and 520 controls). The Scandinavian SCALE study is not included as rs1860661 could not be genotyped in controls using Sequenom. Full size image For all HL combined, two other novel variants at chromosome 3q32 ( CLSTN2 , rs6439924, P =8.3 × 10 −8 , I 2 =0%) and chromosome 7p21 ( ARL4A-ETV1 , rs2058613, P =6.6 × 10 −7 , I 2 =0%) approached genome-wide levels of significance in the discovery set, but were not significant in the replication set ( Supplementary Table 4 ). We used a bioinformatic approach (FunciSNP [18] ) to identify potential functional variants tagged by rs1860661. By querying the 20110521 release of 1,000 genomes database [19] , we identified four SNPs correlated ( r 2 >0.5) with the index SNP (rs1860661). We then extracted publically available ENCODE [20] data on biofeatures, and found that the index SNP rs1860661 and two correlated SNPs, rs10413888 ( r 2 =0.90) and rs8103453 ( r 2 =0.89), map in or near marks of open chromatin and in DNAse hypersensitivity sites in TCF3 in CD20+ B-cell lines. Interestingly, the protective haplotype defined by the minor alleles G-G-G of all three SNPs potentially enhances the efficiency of the binding sites for transcription factors ZBTB7a and E2F1 ( Fig. 5 ). The relative frequencies of each nucleotide (based on a position weight matrix) for the alleles in the ZBTB7A motif of index SNP r1860661 are G:99.8% A:0.2% and for rs10413888 ( r 2 =0.90) are T:0.4% G:97.4%. For rs8103453 ( r 2 =0.89) the E2F1 nucleotide frequencies are A:0% G:97%. 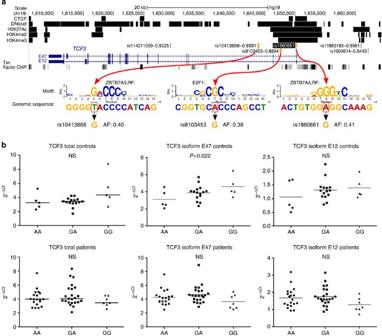Figure 5: Bioinformatic and expression analysis of the TCF3 SNP. (a) Browser view of TCF3 genomic region. Position of ENCODE data for the chromatin biofeatures used to filter correlated SNPs are shown in the top five tracks as black bars. The FunciSNP18analysis track displays correlated SNP positions with the name andr2value. Red arrows highlight the putative functional SNPs for this region. Genomic sequence surrounding the affected SNPs is shown at bottom under the motif-logo of the matched transcription factor, with the risk allele for Hodgkin lymphoma boxed in red. The alternative (protective) allele is displayed next to the SNP name, with allele frequency for Europeans in 1,000 genomes19. (b) TCF3 expression levels determined on RNA isolated from lymphoblastoid cell lines generated by transformation of blood B cells obtained from healthy controls (n=25) and post-therapy Hodgkin lymphoma (n=49) patients, using qRT–PCR. Linear models were used to assess correlation between genotype and TCF3 expression levels. Figure 5: Bioinformatic and expression analysis of the TCF3 SNP. ( a ) Browser view of TCF3 genomic region. Position of ENCODE data for the chromatin biofeatures used to filter correlated SNPs are shown in the top five tracks as black bars. The FunciSNP [18] analysis track displays correlated SNP positions with the name and r 2 value. Red arrows highlight the putative functional SNPs for this region. Genomic sequence surrounding the affected SNPs is shown at bottom under the motif-logo of the matched transcription factor, with the risk allele for Hodgkin lymphoma boxed in red. The alternative (protective) allele is displayed next to the SNP name, with allele frequency for Europeans in 1,000 genomes [19] . ( b ) TCF3 expression levels determined on RNA isolated from lymphoblastoid cell lines generated by transformation of blood B cells obtained from healthy controls ( n =25) and post-therapy Hodgkin lymphoma ( n =49) patients, using qRT–PCR. Linear models were used to assess correlation between genotype and TCF3 expression levels. Full size image To investigate the function of rs1860661, we measured the expression levels of TCF3 , and its two alternative transcripts, E12 and E47, in lymphoblastoid cell lines (LCLs) derived from circulating normal B cells from 49 post-therapy HL patients and 25 unaffected controls using linear models to assess correlation between genotype and TCF3 expression levels ( Fig. 5 ). There was little evidence for correlation with TCF3 expression levels in this small sample, with only a weak association observed in LCLs from controls with the TCF3 -E47 isoform ( P =0.02), whose transcription start site is located close to rs1860661 ( Fig. 5 ). Similarly, there was little evidence in public databases [21] that rs1860661 acts as a TCF3 eQTL, although eQTLs for the two isoforms were not available. Evidence for downregulation of both TCF3 isoforms was observed in seven HL-derived cell lines compared with germinal centre B cells sorted from three different tonsils ( P t -test <0.05) ( Supplementary Fig. 4 ). Exome sequencing of the same set of seven HL cell lines identified a TCF3 missense mutation, p.N551K, ( Supplementary Fig. 4 ) which has also been observed in Burkitt lymphoma [22] . Finally, we selected the subset of 21,608 SNPs included in our GWAS previously identified as cis-eQTLs in B cells alone or both B cells and monocytes [23] . Within this subset, the genomic inflation factor ( λ ) was estimated as 1.16 ( Supplementary Table 5 , Supplementary Fig. 5 ). A λ of 1.16 was not observed within any of 1,000 random draws of 21,608 SNPs of similar minor allele frequency (MAF) taken from the complete HL meta-analysis, ( Supplementary Table 5 ), suggesting a relative overrepresentation of associated variants within this subgroup. In this meta-analysis of 1,816 HL cases and 7,877 controls, we have identified a new susceptibility locus for HL at 19p13.3 in the TCF3 gene and noted associations with previously identified loci at 2p16— REL , 5q31— IL13 , 6p21—HLA region, 8q24 and 10p14— GATA3 . TCF3 is essential for the commitment of lymphoid progenitors to both B-cell and T-cell lineage development [24] , [25] , [26] . In B cells, homodimers of the E47 isoform of TCF3 lead to transcriptional activation of TCF3 target genes including the B cell-specific transcription factors Oct-2 , PU.1 and Bob.1 (ref. 25 ). A molecular and phenotypic hallmark of cHL is the loss of B-cell signature in HRS cells, including lack of the B-cell receptor, and the lineage markers CD19 and CD20. This loss has been attributed to downregulation of Oct-2 , PU.1 and Bob.1 as a consequence of decreased formation of TCF3 -E47 homodimers due to an increased expression of ABF-1 and ID2 , two proteins that bind to and inhibit TCF3 (refs 26 , 27 , 28 ). However, it is also possible that decreased transcription of the TCF3 gene contributes. Renne et al . [26] reported lower average levels of TCF3 expression in cHL-derived cell lines compared with B-cell lines, and we observed significantly lower levels of both TCF3 splice variants in cHL-derived cell lines compared with sorted tonsillar germinal centre B cells. These observations are consistent with the hypothesis that higher TCF3 levels in HRS precursor cells may lead to enhanced retention of the B-cell phenotype, thereby conferring a protective effect for HL. A biofeature analysis suggests that rs1860661 is located in a transcription factor binding site; however, further study is necessary to determine whether rs1860661 is a causal SNP and associated with a true biological effect on TCF3 expression. Interestingly, in one out of seven HL cell lines, we observed a p.N551K missense TCF3 mutation, a mutation also found in Burkitt lymphoma samples [22] , suggesting that investigation of such mutations in HRS cells may be warranted. As expected, previously published subtype (histology) and subgroup (tumour EBV status) associations with SNPs in 2p16, 5q31, 6p31.2, 8q4 and 10p14 regions were observed [11] , [12] , [13] , although at higher significance levels due to the increased power of the meta-analysis, supporting the proposition that cHL is aetiologically heterogeneous. There are clear associations between HLA class I loci and risk of both EBV-positive HL and MCHL, and between HLA class II, IL13 , REL and GATA3 loci and risk of both EBV-negative HL and NSHL. Our data are inconclusive at this time regarding subset heterogeneity for rs1860661. Thus, our data suggest a link between the 19p13.3 locus, including TCF3 , and HL risk. Although we did not demonstrate functionality of rs1860661, it is located in a gene that is known to be downregulated in HL and thus merits further study. Because HL is a rare cancer, amassing substantial numbers of patients for a GWAS study is difficult. Nevertheless, our meta-analysis increased the ability to detect additional loci, to the level of an OR of 1.25 for a MAF of 30% with 80% power, in line with other meta-GWAS. Even so, we considered the potential for the existence of additional risk HL alleles by assessing the evidence for association within genetic variants linked with gene expression levels in B-cell lymphocytes (eQTLs) [23] compared with unselected genetic variants. The existence of additional, as yet unidentified risk variants for HL is suggested by the observation that eQTLs were enriched among the top associations with HL as compared with non-eQTLs ( Supplementary Table 5 ). Ethics All studies were approved by the following human subjects protection committees at the respective institutions: The University of Southern California Institutional Review Board, The Mayo Clinic Institutional Review Boards, The WHO International Agency for Research on Cancer Human Subjects Committee, The University of Chicago Institutional Review Board, Ethics Committees of Dijon and Lyon University Hospitals, Medical Ethical Review Committee of the UMCG, The Regional Ethical Review Board in Stockholm, The Scientific Ethics Committee for the Capital Region of Copenhagen, Research Ethics Committee for Wales 08/MRE09/72, West of Scotland Research Ethic Committee REC4 09/S0704/73, Multi-Centre Research Ethics Committee for Scotland 06/MRE00/83 and the Northern & Yorkshire Regional Ethics Committee. All patients and replication controls signed informed consent. De-identified publically available GWAS data were obtained for the control comparisons in the three-discovery-set GWAS. Source of subjects and GWAS discovery The discovery of meta-analysis was undertaken by two centres (IARC and USC) and was based on summary data from three previously reported GWAS providing genotype data on 1,816 HL cases and 7,877 controls of European descent: The European Collaborative GWAS [12] and The University of Southern California (USC) [13] /University of Chicago (UC) [14] GWAS studies were combined for a single meta-analysis. The European Collaborative GWAS, presented elsewhere [12] , included 1,241 HL cases aged 13–80 (median age=33 years) from five European-based HL studies and 5,726 generic controls aged 17–94 (mean age=62) used in the initial GWAS scan. In addition to the cHL cases described in the initial GWAS, 41 non-cHL cases were also included in the total. The distribution of cases among the five European-based HL studies is as follows: The EPILYMPH Study ( N =196) [29] , the Scotland and Newcastle Lymphoma Group and the Young Adult Hodgkin Disease Case–Control Study ( N =397) [30] , The Scandinavian Lymphoma Aetiology Study (SCALE) ( N =344) [31] , [32] and the Northern Dutch Hodgkin Lymphoma Study ( N =304) [33] . The distribution of the controls by study is as follows: Alcohol-Related Cancers and Genetic Susceptibility in Europe Study ( N =323) [34] ; The International Agency for Research on Cancer Central Europe Study ( N =443) [35] ; The Pancreatic Cancer Cohort Consortium ( N =321) [36] ; The Nijmegen Biomedical Study ( N =1,769) [37] and The Wellcome Trust Case–Control Consortium ( N =2870) [38] . Cases were genotyped at the Centre National de Génotypage using the Illumina Infinium Human660-Quad BeadChip (Illumina San Diego, CA). Multiple sources of generic controls were genotyped on compatible Illumina BeadChips platforms. The USC HL GWAS included 366 European-origin cases (from an original 380) from four sources, (age range 7–58, mean age=29.5); 233 patients, diagnosed <45 years of age between 2000 and 2008, were ascertained from two California SEER registries [13] , and 133 patients, diagnosed between the ages of 7 and 58 from 1975 through 2006, were ascertained from two USC twin registries: the population-based California Twin Program and volunteer International Twin Study [7] , [39] . Of the 366 HL cases, 251 (69%) were diagnosed as NSHL; 72 (20%) as MCHL; 11 (3%) as other cHL; 11 (3%) as lymphocyte predominant HL; and 21 (5%) as not specified. Of the 129 specimens tested for EBV by in situ hybridization [40] , 107 (83%) were negative and 22 (17%) were positive. 90% of the NSHL and 50% of the mixed cellularity tumours were EBV negative. Fourteen cases from the original analysis [13] were removed due to additional QC measures. Controls were 1,137 (from an original 1,142) European-origin females aged 25–42 who were breast cancer controls in the Cancer Genetic Markers and Susceptibility Project (CGEMS) [41] , [42] . USC cases were genotyped using the Illumina 610 Quad BeadChip and controls were genotyped using the Illumina HumanHap550 (v.1.1). The third GWAS was conducted at UC [14] , in which cases consisted of 209 (from an original 214) HL patients diagnosed prior to age 21 (mean age=16) who were participants in the Children’s Cancer Survivor Study, a retrospective study of 14,358 survivors of childhood cancer diagnosed before 21 years of age and surviving at least five years [43] . Of these, 142 (68%) were diagnosed as NSHL and 18 (9%) as MCHL. Five cases from the original analysis [14] were removed due to additional QC measures. Tumour EBV status was not available. Controls were 1,014 (from an original 1,016) cancer-free individuals of European ancestry (464 males and 550 females) from the Genetic Association Informative Network schizophrenia study cohort (phs000021.v1.p1) [44] . Cases were genotyped at UC on the Affymetrix Genome-Wide Human SNP Array 6.0. Permission was obtained for use of CGEMS and GAIN results from dbGAP (dbgap. ncbi.nlm.nih.gov/aa/ dbgap) [41] . Stringent quality control was performed on the genome-wide genotypes by each of the three GWAS centres that conducted a GWAS based on standard procedures [12] , [13] , [14] . To refine associations with previously reported loci and to identify new disease loci, we imputed untyped genotypes using IMPUTE2 (refs 15 , 45 ) and HapMap Phase III ( http://hapmap.ncbi.nlm.nih.gov ) reference genotypes for the USC and UC HL GWAS data and minimac [15] , [46] software and 1000 Genome Project data release 2010–08 reference genotypes [19] for the European Collaborative GWAS [12] . Poorly imputed SNPs, defined by an r 2 <0.30 with MACH1 (ref. 46 )/minimac [15] or an information measure (Is) <0.30 with IMPUTE2 (ref. 33 ), were excluded from the analyses. Each GWAS study used a 10% threshold for missingness. Technical validation of the three novel SNPs with genome-wide significance was performed in the IARC European Collaborative GWAS (300 discovery set case samples and 90 HapMap Ceu Samples) and USC GWAS (36 discovery case samples) using the same TaqMan probes. Concordance for rs1860661, rs6439924 and rs2058613 across GWAS and replication genotyping platforms was between 99.6% for the European Collaborative GWAS and 100% for the USC GWAS. Replication series and genotyping Novel SNP associations were further validated in an independent replication series comprising 1,281 cases and 3,218 control subjects from multiple case–control or case series. DNA from the European subjects was genotyped at the Centre National Genotypage (1,047 HL cases and 2,995 controls from four contributing studies, mean age=42). The EPILYMPH replication set included 64 cases aged 18–78 at diagnosis and 141 controls aged 18–81 from the Czech Republic, France, Germany, Ireland, Italy and Spain [29] ; the French replication series included 366 cases aged 15–93 at diagnosis from a prospective biologic study carried out by LYSA (Lymphoma Study Association) [47] and 1696 French controls genotyped by the Centre National Genotypage (CNG Evry, France); the UK replication series included 499 cases aged 15–90 at diagnosis and 520 controls aged 16–87 at participation from the ELCCS (York) case–control study [48] , the Scotland and Newcastle Epidemiological Study of Hodgkin’s disease [30] and the Young Adult Hodgkin’s Disease Case–Control Study; and the Scandinavian Lymphoma Aetiology Study (SCALE) replication series included 118 cases aged 18–75 and 638 controls aged 19–75 from Sweden and Denmark [31] , [32] , not included in the discovery GWAS. The Mayo Clinic Replication series included 234 cases ages 18–89 at diagnosis and 223 internal medicine or family medicine clinic controls seen for routine appointments [49] (mean age of Mayo Clinic cases and controls=44 years), genotyped at the Molecular Genomics Core of USC. A subset of European controls was also genotyped at the Centre National Genotypage using the Illumina Sentrix HumanHap300 BeadChip (French controls, n =1,696) or Sequenom (SCALE [31] controls, n =638). A TaqMan Pre-Designed SNP Genotyping Assay Mix (containing probes and primers) was used for each SNP (Applied Biosystems, Carlsbad, CA, assay-on-demand order code C__32302340_10 for rs6439924 and C__11969900_10 for rs1860661). No assay could be designed for rs2058613 and therefore a proxy variant ( R 2 =1.0, D′=1.0 in CEU) rs6946457 (assay C__2678118_10) was genotyped. Similarly, rs1860661 could not be genotyped by Sequenom in the SCALE [31] controls as this assay was not able to be designed for this platform. The performance of the assays was validated at the Centre National Genotypage by re-genotyping CEU HapMap samples (US residents with Northern and Western European ancestry) and comparing the results to HapMap genotypes ( http://hapmap.ncbi.nlm.nih.gov ) (IARC) and by re-genotyping 32 samples from the GWAS and comparing the results to the array based genotypes (USC). Within the study samples, duplicate genotyping concordance was greater than 99%. Statistical analysis All calculations were performed using PLINK [50] ( http://pngu.mgh.harvard.edu/~purcell/plink ), SAS version 9.2 (SAS Institute, Cary, NC, USA) and R15.1 (R project). LocusZoom [51] was used for regional visualization of results. LD statistics were calculated based on HapMap3 release 2 using SNAP Proxy Search [52] . In each of the three discovery GWAS analyses, quality control included removal of individuals with cryptic relatedness and a genotyping call rate of <0.95. In addition, SNPs with a call rate of <0.95, a MAF of <0.01 in the data, deviation from Hardy–Weinberg equilibrium ( P <1 × 10 −5 ), or whose genotypes resulted from artifacts were removed. Associations between SNP genotypes and HL risk were evaluated under a log-additive model of inheritance adjusting for sex, study centre (European Collaborative GWAS only) and significant principal components to control for population stratification [53] . A meta-analysis using a fixed effects model weighted on the inverse of the variance was conducted based on GWAS summary statistics for the log-additive model of inheritance [54] . Only variants available in all three GWAS studies, successfully genotyped/imputed, with no evidence of ambiguous strand calls between studies, were included. We examined overdispersion using P -values from the meta-analysis to generate Quantile–Quantile plots and estimate an inflation factor λ , calculated as a ratio of the median of the observed λ 2 statistics for association from the Wald tests over the median (=0.455) of the λ 2 distribution with 1 df [54] ( Supplementary Figs 1 and 2 ). The HLA region was excluded when calculating the λ to reduce the inflation due to numerous SNPs in LD capturing this previously known locus. Associations between the risk alleles and HL and subtypes were assessed using logistic regression to estimate ORs and 95% CIs and P -values within individual studies. Cochran’s Q -statistic to test for heterogeneity and the I 2 statistic to quantify the proportion of the total variation due to heterogeneity was calculated. Fixed-effect values ⩾ 75% are considered the characteristic of large heterogeneity and corresponding variants were excluded from the analysis. Replication analyses were conducted using logistic regression to estimate ORs, 95% CIs and P -values within individual studies. Study-specific estimates were summarized using a meta-analysis procedure as described above. FunciSNP functional annotation To integrate chromatin biofeature annotations with 1000 Genomes [19] genotyping data, we used an in-house developed R package FunciSNP [18] , available at www.Bioconductor.org . We selected publicly available data sets relevant to the development of the B-cell lineage and thus the following ENCODE data sets were employed to filter correlated SNPs that lie within putative enhancer regions with Gene Expression Omnibus accession IDs: B cells CD20+ RO01778 DGF Peaks (GSM1014525), B cells CD20+ RO01778 DNaseI HS Peaks (GSM1024765, GSM1024766), B cells CD20+ RO01794 HS Peaks (GSM1008588), CD20+ (RO 01778) H3K4me3 Histone Mod chromatin immunoprecipitation (ChIP)-seq Peaks (GSM945229), CD20+ RO01794 H3K27ac Histone Mods by ChIP-seq Peaks (GSM1003459), CD20+ (RO01794) H3K4me3 Histone Mod ChIP-seq Peaks (GSM945198), CD20+ CTCF Histone Mods by ChIP-seq Peaks (GSM1003474), CD20+ H2A.Z Histone Mods by ChIP-seq Peaks (GSM1003476), CD20+ H3K4me2 Histone Mods by ChIP-seq Peaks (GSM1003471). To define other physical map features (transcription start sites, 5′UTR, 3′UTR), we downloaded annotations from the February 2009 release of the human genome (GRCh37/hg19) available from the UCSC genome browser [55] . Finally, we used the highly conserved set of predicted targets of microRNA targeting at www.mircode.org (miRcode 11, June 2012 release), and conserved high-quality microRNA target species from www.microRNA.org (June 2010 release). FunciSNP [18] was run with the following settings: a window size of 1 Mb around the index SNP was used with r 2 >0.5. To determine whether FunciSNP-generated SNPs potentially affect the binding of known transcription factors, position-specific weight matrices were employed from Wang et al . [56] To distinguish between neutral and potentially damaging (or activating) variants, both alleles of the SNP were scored by adding up the total matrix score of each of 119 transcription factor motifs for each of the possible start sites in a window around the SNP and flagging the start positions that surpassed a threshold of 80% of the maximum score for each motif. In addition, the scoring was weighted by the difference between maximum and minimum score at each position, so that unconserved and noncritical sites did not influence the score. SNPs that were found within the binding sites of 80% maximum or better were reported along with the score of the alternate allele. A quality score derived from the ratio of the difference in scores/1− (maximum allelic binding to the TF at that position) was used to rank the SNPs and classify them as neutral, damaging or activating. TCF3 expression experiments LCLs were generated from blood samples collected from 74 individuals, including 25 healthy controls and 49 post-therapy cHL patients (from blood samples collected at least 1 year after completion of all therapies) by infection of PBMCs with the EBV strain B95-8. Genotyping of the LCLs was carried out using a TaqMan SNP assay. Expression levels were assessed using quantitative reverse transcriptase PCR which was performed on all cell lines using the TCF3 assay and isoform-specific primer sets. Association between TCF3 gene expression levels and TCF3 genotype was assessed by linear regression, separately for cHL cases and controls, using PLINK [50] . To compare TCF3 expression in cHL cell lines to normal tonsillar germinal centre B cells, germinal centre B cells were sorted from three independent tonsils (CD19+CD38+IgD−). HL-derived cell lines, that is, L428, L540, L591, L1236, KM-H2, SUPHD1 (available from Braunschweig, Germany) and DEV (A. van den Berg Laboratory) [57] , were cultured in RPMI 1640 medium (Lonza Walkersville, Walkersville, MD) supplemented with 5–20% fetal calf serum, 100U ml −1 penicillin/streptomycin and ultraglutamine (Lonza Walkersville) in a 5% CO 2 atmosphere at 37 °C. DNA isolation and genotyping (TaqMan SNP assay, C_11969900_10) was carried out using standard procedures. RNA was isolated using Trizol (Invitrogen, Carlsbad, USA) and DNAse treated (Ambion, Foster City, CA). The RNA concentration was measured with a NanodropTM 1000 Spectrophotometer (Thermo Fisher Scientific, Waltham, USA) and integrity was evaluated by the Experion system. cDNA was synthesized using 500 ng input RNA, Superscript II and random primers according to the manufacturer’s protocol (Invitrogen). quantitative reverse transcriptase PCR was performed on all samples using the TCF3 assay and isoform-specific primer sets in triplicate. Relative expression levels were calculated using TBP as housekeeping gene and data were expressed as the 2-deltaCt values. A t -test was used to test for TCF3 expression level differences in cHL cell lines compared with germinal centre B cells. TCF3 mutation analysis In an ongoing whole-exome sequencing analysis, we noted a missense mutation (p.N551K) in the TCF3 gene in one out of seven HL-derived cell lines, that is, SUPHD1. To confirm the presence of the mutation and expression of the mutant allele, we amplified cDNA of the SUPHD1 cell line by PCR with AmpliTaq Gold DNA Polymerase, PE Buffer II and MgCl 2 (Applied Biosystems) and primers designed for the region of interest (Primer Express, Applied Biosystems). Primers were ordered with an M13-tail (underlined), to allow direct sequencing of the PCR product (forward 5′- gtaaaacgacggccagt cggaggaggagaagaaggag-3′ and reversed 5′- ggaaacagctatgaccatgg cttggtctgcgctttgtc-3′). PCR products were run on an agarose gel to check efficiency and purified by high pure PCR product purification kit (Roche, Mannheim, Germany) and sent for sequencing (LGC Genomics). HL GWAS genetic variants in eQTLs From the HL GWAS meta-analysis, we selected a subset of genetic variants that were (cis) eQTLs in (B cells alone or both B cells and monocytes), based on Fairfax et al . [23] Variants located within the HLA region (Position 6:25,000,000 to 6:35,000,000) were excluded due to the very high degree of LD, leaving 21,608 SNPs. We used a permutation procedure to consider the range of λ expected by chance by randomly drawing 1,000 subsets (with replacement) of 21,608 SNPs taken from the complete HL meta-analysis 885,168 non-MHC genetics variants of the original HL meta-analysis. We then estimated λ within each of randomly selected 1,000 subsets of 21,608 SNPs. How to cite this article : Cozen, W. et al . A meta-analysis of Hodgkin lymphoma reveals 19p13.3 TCF3 as a novel susceptibility locus. Nat. Commun. 5:3856 doi: 10.1038/ncomms4856 (2014). Accession codes : Exome sequence data for the TCF3 gene in 7 Hodgkin lymphoma cell lines has been deposited in the EMBL European Bioinformatics Institute database under the accession code PRJEB5699 (or ERP005119).